Protein kinase D1 drives pancreatic acinar cell reprogramming and progression to intraepithelial neoplasia The transdifferentiation of pancreatic acinar cells to a ductal phenotype (acinar-to-ductal metaplasia, ADM) occurs after injury or inflammation of the pancreas and is a reversible process. However, in the presence of activating Kras mutations or persistent epidermal growth factor receptor (EGF-R) signalling, cells that underwent ADM can progress to pancreatic intraepithelial neoplasia (PanIN) and eventually pancreatic cancer. In transgenic animal models, ADM and PanINs are initiated by high-affinity ligands for EGF-R or activating Kras mutations, but the underlying signalling mechanisms are not well understood. Here, using a conditional knockout approach, we show that protein kinase D1 (PKD1) is sufficient to drive the reprogramming process to a ductal phenotype and progression to PanINs. Moreover, using 3D explant culture of primary pancreatic acinar cells, we show that PKD1 acts downstream of TGFα and Kras, to mediate formation of ductal structures through activation of the Notch pathway. Approximately 95% of all pancreatic ductal adenocarcinoma (PDAC) express either somatic activating mutations of Kras [1] or show increased epidermal growth factor receptor (EGF-R) signalling [2] , [3] . A pathological progression model for PDAC suggests that it originates from a duct-like progenitor cell type that gives rise to pancreatic intraepithelial neoplasia (PanIN) [4] , [5] , [6] . The use of genetic animal models provided evidence that most differentiated pancreatic epithelial cell types, including acinar cells, can transdifferentiate to the duct-like cell type that generates PanIN lesions [7] , [8] , [9] . Acinar-to-ductal metaplasia (ADM) is accompanied by altered gene expression including a decrease in acinar markers such as amylase or carboxypeptidase A, or Mist-1 (ref. 10 ), and the acquisition of ductal markers such as cytokeratin-19 (CK-19) or mucin-1 (ref. 11 ). However, cells that undergo ADM also show increased expression of Pdx1 (pancreatic and duodenal homeobox-1) [12] and the Notch targets Hes-1 (hairy and enhancer of split 1) and Hey-1 (hairy enhancer of split-related with YRPW motif protein-1) [13] , indicating that this reprogramming process also leads to a less-differentiated, immature pancreatic cell type [5] . Mediators of ADM in vivo are activating mutations of Kras, inflammation and persistent activation of the EGF-R. For example, transgenic expression of the EGF-R ligand transforming growth factor-α (TGFα) under the control of the elastase promoter can induce pancreatic metaplasia [14] . Moreover, in a transgenic animal model, in which an oncogenic mutant of Kras is expressed in acinar cells of the pancreas, ADM and progression to PanIN lesions are observed [7] . These events caused by mutated Kras are further potentiated and lead to pancreatic cancer, when additional pancreatic inflammation occurs [15] , [16] , [17] , [18] . Although such genetic animal models are ideal to provide insight into the contribution of molecules to organ pathology, such long-term studies make it difficult to investigate actual signalling mechanisms involved in the ADM process. Signalling mechanisms that regulate the acinar–ductal transformation process can be studied in an ex vivo explant three-dimensional (3D) cell culture model in which primary acinar cells are isolated from the pancreas and transdifferentiated in the presence of growth factors. For example, the EGF-R ligands TGFα and EGF can drive ADM in vitro [19] , [20] , [21] , [22] , [23] . Using a 3D explant model, and either PKD inhibitors or a PKD1 knockdown approach, we here provide evidence that the serine/threonine kinase protein kinase D1 (PKD1) is necessary for TGFα- and Kras-mediated formation of duct-like structures originating from acinar cells. Moreover, we show that active PKD1 is sufficient to drive this transdifferentiation process and confirm the relevance of this signalling pathway in vivo , as the knockout of PKD1 in acinar cells of p48 cre ;Kras G12D mice decreases the progression of ADM to PanIN lesions. As acinar cell transformation and progression to PanIN lesions is one of the earliest known events contributing to the development of pancreatic cancer, our data suggest that pharmacologic inhibition of PKD may be an effective strategy to prevent early changes involved in development of pancreatic cancer. PKD1 is upregulated in transforming acinar cells Transformation of acinar cells to a duct-like phenotype and formation of PanINs can be observed in vivo in transgenic animals expressing TGFα or constitutively active Kras [5] , [14] , [16] , [24] , [25] . Of the three PKD isoforms, PKD1, PKD2 and PKD3, acinar cells of normal pancreas only express PKD3 ( Supplementary Fig. 1a and ref. 26 ). However, in transgenic mice that express TGFα in the pancreatic epithelium, in areas where acinar cells undergo ADM, the PKD expression pattern was altered ( Fig. 1a ). PKD1 showed increased expression in regions of ADM and PanIN lesions, but not in adjacent regions of ‘normal’ acinar structures ( Fig. 1A4 ). Of note, the cells forming these ‘normal’ acinar structures also express the TGFα transgenic allele, but have not yet undergone transformation. The other two PKD isoforms, PKD2 and PKD3, were expressed in the more ‘normal’ acinar structures of the TGFα transgenic mice, but in contrast to PKD1, their expression decreased in regions of ADM ( Fig. 1A5 , A6 ). Upstream activating phosphorylations of PKD in regions of ADM was determined by immunohistochemistry (IHC) with a phosphospecific antibody that specifically recognizes PKD phosphorylated at the activation loop (labelled: anti-pS744/748-PKD). This antibody does not distinguish between PKD1, PKD2 and PKD3. However, staining with this antibody overlapped with PKD1 staining ( Fig. 1A3 ), indicating that in ADM regions PKD1 is upregulated and phosphorylated by its upstream kinases. At a later age, these mice developed more significant areas of ADM and PanINs, which exhibited even more significant elevation in PKD1 expression ( Fig. 1b ). 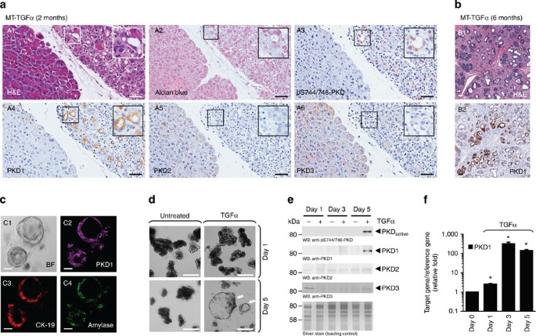Figure 1: PKD1 is upregulated in pancreatic acinar cells undergoing ADM. (a,b) Pancreatic tissue (normal acinar area and regions with ADM and PanINs) from MT-TGFα transgene mice was stained with haematoxylin and eosin (H&E), Alcian Blue, or analysed by IHC for expression of PKD1 (anti-PKD1), PKD2 (anti-PKD2), PKD3 (anti-PKD3), or active PKD activity (anti-pS744/748-PKD), as indicated. Scale bar, 50 μm. (c) Primary acinar cells were isolated from mouse pancreas and seeded in 3D culture in phenol red-free, growth factor-containing Matrigel. At day 5, expression of PKD1 (anti-PKD1, deep red), CK-19 (ductal marker, red) and amylase (acinar cell marker, green) were analysed by immunofluorescence. BF, bright field. Scale bar, 50 μm. (d–f) Primary acinar cells were isolated from mouse pancreas, seeded in 3D culture in collagen and transdifferentiation was induced with TGFα (50 ng ml−1) as indicated. Ducts formed were photographed (d, Scale bar, 100 μm), isolated from the collagen and analysed by western blotting for expression of PKD1, PKD2, PKD3 and active PKD (anti-S744/748-PKD) as indicated (e), or analysed by quantitative PCR for PKD1 expression (f). Ine, silver staining served as loading control. In (f, * indicates statistical significance (P<0.05; Student’st-test) as compared with control. Error bars (s.d.) were obtained from three experimental replicates. All experiments shown were performed at least three times with similar results. Figure 1: PKD1 is upregulated in pancreatic acinar cells undergoing ADM. ( a , b ) Pancreatic tissue (normal acinar area and regions with ADM and PanINs) from MT-TGFα transgene mice was stained with haematoxylin and eosin (H&E), Alcian Blue, or analysed by IHC for expression of PKD1 (anti-PKD1), PKD2 (anti-PKD2), PKD3 (anti-PKD3), or active PKD activity (anti-pS744/748-PKD), as indicated. Scale bar, 50 μm. ( c ) Primary acinar cells were isolated from mouse pancreas and seeded in 3D culture in phenol red-free, growth factor-containing Matrigel. At day 5, expression of PKD1 (anti-PKD1, deep red), CK-19 (ductal marker, red) and amylase (acinar cell marker, green) were analysed by immunofluorescence. BF, bright field. Scale bar, 50 μm. ( d – f ) Primary acinar cells were isolated from mouse pancreas, seeded in 3D culture in collagen and transdifferentiation was induced with TGFα (50 ng ml −1 ) as indicated. Ducts formed were photographed ( d , Scale bar, 100 μm), isolated from the collagen and analysed by western blotting for expression of PKD1, PKD2, PKD3 and active PKD (anti-S744/748-PKD) as indicated ( e ), or analysed by quantitative PCR for PKD1 expression ( f ). In e , silver staining served as loading control. In ( f , * indicates statistical significance ( P <0.05; Student’s t -test) as compared with control. Error bars (s.d.) were obtained from three experimental replicates. All experiments shown were performed at least three times with similar results. Full size image Figure 5: PKD1 mediates formation of duct-like structures through Notch. ( a ) Scatter plot showing fold changes in expression of genes in control primary acinar cells or cells expressing constitutively active PKD1 (PKD1.CA). The centre line indicates no difference between the expression of genes under both conditions. 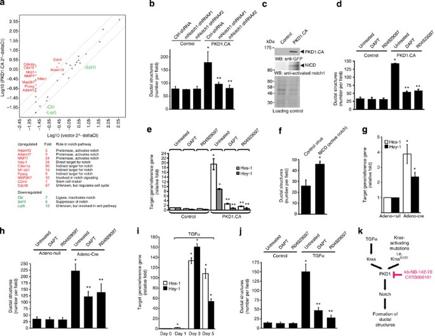Figure 5: PKD1 mediates formation of duct-like structures through Notch. (a) Scatter plot showing fold changes in expression of genes in control primary acinar cells or cells expressing constitutively active PKD1 (PKD1.CA). The centre line indicates no difference between the expression of genes under both conditions. The side lines indicate a fourfold difference in either direction. The genes expressed more than fourfold in the PKD1.CA group as compared with the control group are labelled in red. The genes expressed lower than fourfold in the PKD1.CA group are labelled in green. Their role in the Notch pathway as well as fold change is provided in the table. (b) Primary acinar cells were isolated from mouse pancreas and infected with lentivirus harbouring (scrambled) control shRNA (Ctrl-shRNA) or two different sequences of Notch1-shRNA (#1 and #2) specifically targeting mouse Notch1. In addition, cells were lentivirally infected with active PKD1 (PKD1.CA) or control virus as indicated. Cells were then seeded in 3D culture in collagen and formation of ductal structures was quantified. (c) Primary acinar cells were isolated from mouse pancreas and lentivirally infected with control or GFP-tagged active PKD1 (PKD1.CA; PKD1.S738E/S742E mutant). Cells were then seeded in 3D culture in collagen. At day 6, cells were re-isolated and analysed by western blotting for activated Notch 1 fragment (NICD). Expression of PKD1.CA was controlled by western blotting against GFP. Silver staining served as a loading control. (d,e) After isolation and infection with control or PKD1.CA harbouring lentivirus, primary acinar cells were seeded in collagen 3D culture in the absence or the presence of the γ-secretase inhibitors DAPT (5 μM) or RO4929097 (10 nM) as indicated. At day 6, formation of ductal structures was determined (d), or cells were isolated from the collagen and analysed by quantitative PCR for expression of the Notch target genesHes-1andHey-1(e). (f) Primary acinar cells were isolated from mouse pancreas and infected with lentivirus harbouring an active Notch fragment (NICD) or control virus. Cells were then seeded in 3D culture in collagen and formation of ductal structures was quantified. (g,h) Primary acinar cells from LSL-KrasG12Dmice were isolated from mouse pancreas and expression of mutant Kras was induced by adenoviral infection of cre-recombinase as indicated (Adeno-Cre; or Adeno-null as control). Cells then were seeded in collagen 3D culture in the absence or the presence of the γ-secretase inhibitors DAPT (5 μM) or RO4929097 (10 nM) as indicated. At day 6, cells were isolated from the collagen and analysed by quantitative PCR for expression of the Notch target genesHes-1andHey-1(G), and formation of ductal structures was determined (h). (i,j) Primary acinar cells were seeded in collagen 3D culture in the absence or the presence of TGFα (50 ng ml−1) and the γ-secretase inhibitors DAPT (5 μM) or RO4929097 (10 nM) as indicated. At indicated days, cells were isolated from the collagen and analysed by quantitative PCR for expression of the Notch target genesHes-1andHey-1(i), and formation of ductal structures was determined (j). In all figures shown inb,d–j, * indicates statistical significance (P<0.05; Student’st-test) as compared with control and ** indicates statistical significance (P<0.05; Student’st-test) as compared with stimulus. Error bars (s.d.) were obtained from three experimental replicates. (k) Schematic of a TGFα- and Kras-induced PKD1-Notch signalling pathway that drives formation of pancreatic duct-like structures and PanIN formation. All experiments shown were performed at least three times with similar results. The side lines indicate a fourfold difference in either direction. The genes expressed more than fourfold in the PKD1.CA group as compared with the control group are labelled in red. The genes expressed lower than fourfold in the PKD1.CA group are labelled in green. Their role in the Notch pathway as well as fold change is provided in the table. ( b ) Primary acinar cells were isolated from mouse pancreas and infected with lentivirus harbouring (scrambled) control shRNA (Ctrl-shRNA) or two different sequences of Notch1-shRNA (#1 and #2) specifically targeting mouse Notch1. In addition, cells were lentivirally infected with active PKD1 (PKD1.CA) or control virus as indicated. Cells were then seeded in 3D culture in collagen and formation of ductal structures was quantified. ( c ) Primary acinar cells were isolated from mouse pancreas and lentivirally infected with control or GFP-tagged active PKD1 (PKD1.CA; PKD1.S738E/S742E mutant). Cells were then seeded in 3D culture in collagen. At day 6, cells were re-isolated and analysed by western blotting for activated Notch 1 fragment (NICD). Expression of PKD1.CA was controlled by western blotting against GFP. Silver staining served as a loading control. ( d , e ) After isolation and infection with control or PKD1.CA harbouring lentivirus, primary acinar cells were seeded in collagen 3D culture in the absence or the presence of the γ-secretase inhibitors DAPT (5 μM) or RO4929097 (10 nM) as indicated. At day 6, formation of ductal structures was determined ( d ), or cells were isolated from the collagen and analysed by quantitative PCR for expression of the Notch target genes Hes-1 and Hey-1 ( e ). ( f ) Primary acinar cells were isolated from mouse pancreas and infected with lentivirus harbouring an active Notch fragment (NICD) or control virus. Cells were then seeded in 3D culture in collagen and formation of ductal structures was quantified. ( g , h ) Primary acinar cells from LSL-Kras G12D mice were isolated from mouse pancreas and expression of mutant Kras was induced by adenoviral infection of cre-recombinase as indicated (Adeno-Cre; or Adeno-null as control). Cells then were seeded in collagen 3D culture in the absence or the presence of the γ-secretase inhibitors DAPT (5 μM) or RO4929097 (10 nM) as indicated. At day 6, cells were isolated from the collagen and analysed by quantitative PCR for expression of the Notch target genes Hes-1 and Hey-1 (G), and formation of ductal structures was determined ( h ). ( i , j ) Primary acinar cells were seeded in collagen 3D culture in the absence or the presence of TGFα (50 ng ml −1 ) and the γ-secretase inhibitors DAPT (5 μM) or RO4929097 (10 nM) as indicated. At indicated days, cells were isolated from the collagen and analysed by quantitative PCR for expression of the Notch target genes Hes-1 and Hey-1 ( i ), and formation of ductal structures was determined ( j ). In all figures shown in b , d – j , * indicates statistical significance ( P <0.05; Student’s t -test) as compared with control and ** indicates statistical significance ( P <0.05; Student’s t -test) as compared with stimulus. Error bars (s.d.) were obtained from three experimental replicates. ( k ) Schematic of a TGFα- and Kras-induced PKD1-Notch signalling pathway that drives formation of pancreatic duct-like structures and PanIN formation. All experiments shown were performed at least three times with similar results. Full size image To investigate a potential role for PKD isoforms in ADM, we next used an established explant model [22] , [23] in which mouse primary pancreatic acinar cells are isolated and then reseeded ex vivo in 3D cell culture in Matrigel (extracellular matrix) to induce ADM. Duct-like structures formed after 5 days in culture showed expression of PKD1 as well as markers for both acinar cells (amylase) and ductal cells (CK-19), indicating their transdifferentiated or progenitor phenotype ( Fig. 1c ). PKD1 expression was observed only in freshly developed ducts, but not in remaining acinar cells ( Supplementary Fig. 1b , top). Moreover, PKD was active in newly formed ducts ( Supplementary Fig. 1b , bottom). Thus, data obtained with this ex vivo model are in accordance with our in vivo data. Next, we used a more defined explant model in which acinar cells are seeded in collagen I 3D culture and transdifferentiation is induced by TGFα [23] , [27] . Primary acinar cells from mouse pancreas seeded in collagen undergo full ADM within ~5 days, when treated with TGFα ( Fig. 1d ). This was accompanied by increased PKD1 protein expression, whereas PKD2 and PKD3 were marginally or not expressed at days 3 and 5 ( Fig. 1e ). Increased expression of PKD1 correlated with a corresponding increase in PKD activity ( Fig. 1e ), as well as a decrease in acinar markers and an increase in ductal markers, such as amylase or CK-19, respectively ( Supplementary Fig. 1c ). Of note, short-term stimulation (up to 5 h) of acinar cells with TGFα did not result in upregulation of PKD1 protein or activity ( Supplementary Fig. 1d ). Indeed, cells undergoing transdifferentiation to a duct-like phenotype showed up to 400-fold induction of PKD1 messenger RNA at days 3 and 5 ( Fig. 1f ), suggesting that upregulation of protein is regulated at the mRNA level. PKD is necessary for TGFα-mediated acinar cell metaplasia To determine whether upregulation of PKD1 expression and activity is simply correlative with ADM, or alternatively is causative for the process, we compared TGFα-induced ADM of mouse primary pancreatic acinar cells that were lentivirally infected with control short hairpin RNA (shRNA) or shRNA specifically targeting PKD1. TGFα-induced formation of ductal structures was significantly decreased to ~50% when PKD1 was knocked down ( Fig. 2a ). This was observed with two different shRNA sequences for mouse PKD1 (mPKD1-shRNA#1 and mPKD1-shRNA#2). Moreover, TGFα-mediated effects on ADM were rescued by expression of exogenous human PKD1 that is not affected by the shRNA targeting mouse PKD1. Knockdown of PKD1 not only had effects on the numbers of ducts formed but also affected their size. Depletion of PKD1 expression levels to ~50% ( Supplementary Fig. 2a ) not only led to a 50% reduction of TGFα-induced ADM events ( Fig. 2b , left side) but ducts formed were also smaller in size. For example, in the presence of PKD1-shRNA the average ductal area was 0.001 mm 2 , whereas the average ductal diameter in the control counterparts was 0.0025, mm 2 , as determined by analysing 100 ducts of each condition for their ductal area ( Fig. 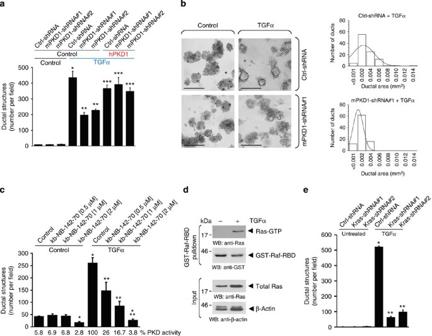2b , right side). Figure 2: PKD is necessary for TGFα-mediated metaplasia to ductal structures. (a,b) Primary acinar cells were isolated from mouse pancreas and infected with lentivirus harbouring (scrambled) control shRNA (Ctrl-shRNA) or two different sequences of PKD1-shRNA (#1 and #2) specifically targeting mouse PKD1. In addition, cells were lentivirally infected with human PKD1 or control virus, as indicated. Cells were then seeded in 3D culture in collagen and transdifferentiation was induced with TGFα (50 ng ml−1). Formation of ductal structures was quantified (a), or ducts formed were photographed and the ductal area of 100 ducts was determined (b). Inb, scale bar, 200 μm. (c) Primary acinar cells were isolated from mouse pancreas, seeded in 3D culture in collagen and transdifferentiation was induced with TGFα (50 ng ml−1) in the absence or the presence of the PKD inhibitor kb-NB-142-70 at indicated doses. ADM events were quantified. (d) Primary acinar cells were isolated from mouse pancreas and stimulated with TGFα (50 ng ml−1, 48 h). Active Ras was pulled down using GST-Raf-RBD. Samples were analysed by SDS–PAGE and immunoblotting for pulled-down active Ras (anti-Ras), GST-Raf-RBD input (anti-GST), as well as other input controls (anti-Ras and anti-β-actin). (e) Primary acinar cells were isolated from mouse pancreas, infected with lentivirus harbouring (scrambled) control shRNA (Ctrl-shRNA) or Kras-shRNA (two different specific sequences, #1 and #2), seeded in 3D culture in collagen and transdifferentiation was induced with TGFα (50 ng ml−1). ADM events were quantified. *Statistical significance (P<0.05; Student’st-test) as compared with control. ** Statistical significance (P<0.05; Student’st-test) as compared with TGFα treatment. *** Statistical significance (P<0.05; Student’st-test) as compared with respective shRNA sample. Error bars (s.d.) were obtained from three experimental replicates. All experiments shown were performed at least three times with similar results. Figure 2: PKD is necessary for TGFα-mediated metaplasia to ductal structures. ( a , b ) Primary acinar cells were isolated from mouse pancreas and infected with lentivirus harbouring (scrambled) control shRNA (Ctrl-shRNA) or two different sequences of PKD1-shRNA (#1 and #2) specifically targeting mouse PKD1. In addition, cells were lentivirally infected with human PKD1 or control virus, as indicated. Cells were then seeded in 3D culture in collagen and transdifferentiation was induced with TGFα (50 ng ml −1 ). Formation of ductal structures was quantified ( a ), or ducts formed were photographed and the ductal area of 100 ducts was determined ( b ). In b , scale bar, 200 μm. ( c ) Primary acinar cells were isolated from mouse pancreas, seeded in 3D culture in collagen and transdifferentiation was induced with TGFα (50 ng ml −1 ) in the absence or the presence of the PKD inhibitor kb-NB-142-70 at indicated doses. ADM events were quantified. ( d ) Primary acinar cells were isolated from mouse pancreas and stimulated with TGFα (50 ng ml −1 , 48 h). Active Ras was pulled down using GST-Raf-RBD. Samples were analysed by SDS–PAGE and immunoblotting for pulled-down active Ras (anti-Ras), GST-Raf-RBD input (anti-GST), as well as other input controls (anti-Ras and anti-β-actin). ( e ) Primary acinar cells were isolated from mouse pancreas, infected with lentivirus harbouring (scrambled) control shRNA (Ctrl-shRNA) or Kras-shRNA (two different specific sequences, #1 and #2), seeded in 3D culture in collagen and transdifferentiation was induced with TGFα (50 ng ml −1 ). ADM events were quantified. *Statistical significance ( P <0.05; Student’s t -test) as compared with control. ** Statistical significance ( P <0.05; Student’s t -test) as compared with TGFα treatment. *** Statistical significance ( P <0.05; Student’s t -test) as compared with respective shRNA sample. Error bars (s.d.) were obtained from three experimental replicates. All experiments shown were performed at least three times with similar results. Full size image As PKD1 protein is very stable and a full knockdown was not achieved, we additionally used the PKD-specific inhibitors kb-NB-142-70 and CRT0066101, to determine the role of PKD activity in the formation of duct-like structures. Treatment of cells with either kb-NB-142-70 ( Fig. 2c ) or CRT0066101 ( Supplementary Fig. 2c ) completely blocked TGFα-mediated ADM in a dose-dependent manner without affecting cell viability ( Supplementary Fig. 2b,c ). Taken together, our results clearly indicate that PKD1 expression and activity are necessary for TGFα-mediated ADM, and contribute to duct formation and size. In transgenic animal models, expression of active Kras in pancreatic cells can drive the formation of ADM and further progression to PanINs or cystic papillary lesions [7] , [28] , [29] . Therefore, we next tested whether TGFα in our ex vivo explant model mediates its effects on ADM through active Ras proteins. Primary acinar cells treated with TGFα (short-term and long-term stimulation) showed an increase in active Ras as measured by pull-down assays using GST-Raf-RBD ( Fig. 2d and Supplementary Fig. 2d ). Such pull-down assays do not distinguish between the Ras isoforms that are activated by TGFα. However, specific knockdown of Kras in acinar cells using two different lentiviral shRNA constructs effectively blocked TGFα-mediated duct formation ( Fig. 2e ). These data suggest that TGFα-induced ADM is mediated, in part, through activation of endogenous Kras. PKD is necessary for Kras-mediated acinar cell metaplasia To further determine the role of PKD1 downstream of active Kras in the ADM process, we analysed bi-transgenic p48 cre ;Kras G12D mice that express mutant Kras in pancreatic epithelial cells for PKD1 expression. We found that expression of PKD1 is upregulated in regions of ADM and in PanINs ( Fig. 3a ). To recapitulate these results in vitro , we isolated acinar cells from LSL-Kras G12D mice and induced the expression of active Kras with an adenovirus harbouring cre recombinase (Adeno-Cre) before the 3D explant culture. Expression of active Kras in acinar cells led to a dramatic increase in ADM events ( Fig. 3b ), as well as upregulation of PKD1 expression and activity, similar to that previously observed in cells treated with TGFα ( Fig. 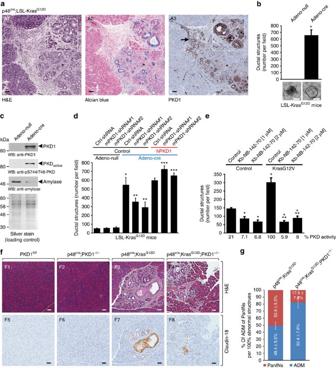3c ). Figure 3: PKD1 is necessary for Kras-induced metaplasia to ductal structures. (a) Pancreatic tissue (normal acinar area and regions with ADM) from bi-transgenic p48cre;KrasG12Dmice was stained with haematoxylin and eosin (H&E), Alcian Blue, or analysed by IHC for PKD1 expression (anti-PKD1). The asterisk shows a typical region of newly formed ductal structures. The arrow shows immune cells staining positive for PKD1. Scale bar, 50 μm. (b,c) Primary acinar cells were isolated from LSL-KrasG12Dmice and infected with Adeno-Cre (or control virus) to induce expression of KrasG12D. Formation of ductal structures was quantified and ducts formed were photographed (b), or ducts formed were isolated and analysed by western blotting for PKD1 expression (anti-PKD1) or activity (anti-pS744/748) and anti-amylase (c). Inb, scale bar, 200 μm; inc, silver staining served as loading control. (d) Primary acinar cells from LSL-KrasG12Dmice were isolated from mouse pancreas and infected with lentivirus harbouring (scrambled) control shRNA (Ctrl-shRNA) or two different sequences of PKD1-shRNA (#1 and #2) specifically targeting mouse PKD1. Expression of mutant Kras was induced by adenoviral infection of cre-recombinase as indicated (Adeno-Cre), or Adeno-null as control. In addition, cells were lentivirally infected with human PKD1 or control virus as indicated. Cells were then seeded in 3D culture in collagen and formation of ductal structures was quantified. (e) Primary acinar cells were isolated from mouse pancreas, lentivirally infected with KrasG12Vand then seeded in 3D culture in collagen in the absence or the presence of the PKD inhibitor kb-NB-142-70 at indicated doses. Formation of ductal structures was quantified. * Statistical significance (P<0.05; Student’st-test) as compared with control. ** Statistical significance (P<0.05; Student’st-test) as compared with stimulus. *** Statistical significance (P<0.05; Student’st-test) as compared with respective shRNA sample. Error bars (s.d.) were obtained from three experimental replicates. (f) Analysis of control, p48cre;KrasG12Dand p48cre;KrasG12D;PKD1−/−mice for regions of ADM/PanIN using H&E staining and IHC for claudin-18. Additional controls are depicted inSupplementary Fig. 3. Scale bar, 50 μm. (g) Quantitation of ADM and PanIN lesions in p48cre;KrasG12Dand p48cre;KrasG12D;PKD1−/−mice. Figure 3: PKD1 is necessary for Kras-induced metaplasia to ductal structures. ( a ) Pancreatic tissue (normal acinar area and regions with ADM) from bi-transgenic p48 cre ;Kras G12D mice was stained with haematoxylin and eosin (H&E), Alcian Blue, or analysed by IHC for PKD1 expression (anti-PKD1). The asterisk shows a typical region of newly formed ductal structures. The arrow shows immune cells staining positive for PKD1. Scale bar, 50 μm. ( b , c ) Primary acinar cells were isolated from LSL-Kras G12D mice and infected with Adeno-Cre (or control virus) to induce expression of Kras G12D . Formation of ductal structures was quantified and ducts formed were photographed ( b ), or ducts formed were isolated and analysed by western blotting for PKD1 expression (anti-PKD1) or activity (anti-pS744/748) and anti-amylase ( c ). In b , scale bar, 200 μm; in c , silver staining served as loading control. ( d ) Primary acinar cells from LSL-Kras G12D mice were isolated from mouse pancreas and infected with lentivirus harbouring (scrambled) control shRNA (Ctrl-shRNA) or two different sequences of PKD1-shRNA (#1 and #2) specifically targeting mouse PKD1. Expression of mutant Kras was induced by adenoviral infection of cre-recombinase as indicated (Adeno-Cre), or Adeno-null as control. In addition, cells were lentivirally infected with human PKD1 or control virus as indicated. Cells were then seeded in 3D culture in collagen and formation of ductal structures was quantified. ( e ) Primary acinar cells were isolated from mouse pancreas, lentivirally infected with Kras G12V and then seeded in 3D culture in collagen in the absence or the presence of the PKD inhibitor kb-NB-142-70 at indicated doses. Formation of ductal structures was quantified. * Statistical significance ( P <0.05; Student’s t -test) as compared with control. ** Statistical significance ( P <0.05; Student’s t -test) as compared with stimulus. *** Statistical significance ( P <0.05; Student’s t -test) as compared with respective shRNA sample. Error bars (s.d.) were obtained from three experimental replicates. ( f ) Analysis of control, p48 cre ;Kras G12D and p48 cre ;Kras G12D ;PKD1 −/− mice for regions of ADM/PanIN using H&E staining and IHC for claudin-18. Additional controls are depicted in Supplementary Fig. 3 . Scale bar, 50 μm. ( g ) Quantitation of ADM and PanIN lesions in p48 cre ;Kras G12D and p48 cre ;Kras G12D ;PKD1 −/− mice. Full size image As previously observed for TGFα, Kras G12D -induced formation of ductal structures was significantly decreased when PKD1 was knocked down using two different shRNA sequences for mouse PKD1 ( Fig. 3d ). Effects on ADM were rescued by ectopic expression of human PKD1 that is not affected by the shRNA targeting mouse PKD1. Lentiviral expression of active TdTomato-tagged Kras (Kras G12V ) in normal acinar cells was also able to drive ADM, albeit less efficiently (we observed only a two- to threefold increase in ADM events; Fig. 3e , compare bars 1 with 4), and this was blocked by pharmacologic inhibition of PKD1 with Kb-NB-142-70 ( Fig. 3e and Supplementary Fig. 3a ). The difference in the extent of ADM events observed in cells from LSL-Kras G12D mice infected with Adeno-Cre virus as compared with cells from normal mice infected with lentivirus harbouring a TdTomato-tagged Kras G12V may be due to the use of primary acinar cells from different pancreata in each experiment, indicating that the adenoviral system is more efficient in targeting acinar cells, or that the fluorescence tag renders Kras less effective in mediating ADM. However, of importance, we show an increase in ADM events using two different approaches, to increase expression of active Kras in pancreatic acinar cells. Taken together, these data suggest that PKD1 acts downstream of active Kras in the ADM process. To test whether the signalling observed in 3D explant culture has relevance in vivo , we compared ADM and PanIN formation in p48 cre ;Kras G12D mice with that in p48 cre ;Kras G12D ;PKD1 −/− mice, or respective controls. The knockout of PKD1 in pancreatic acinar cells significantly decreased Kras G12D -caused formation of PanIN lesions as judged by haematoxylin and eosin staining and IHC for claudin-18 ( Fig. 3f , for additional controls see Supplementary Fig. 3d,f ). Although overall numbers of abnormal structures (ADM and PanINs all combined) were similar ( Supplementary Fig. 3e ), a more detailed analysis showed that the knockout of PKD1 delays the progression of ADM areas to PanINs ( Fig. 3g ). PKD1 drives formation of an immature ductal phenotype Next, we tested whether PKD1 is sufficient to drive the formation of duct-like structures. For this purpose, we infected pancreatic primary acinar cells with a lentivirus expressing either wild-type PKD1, an active mutant (PKD1.CA, PKD1.S738E.S742E) or a kinase-dead version (PKD1.KD, PKD1.K612W). Introduction of wild-type PKD1 increased ADM events in 3D explant cell culture approximately twofold and constitutively active PKD1 approximately sixfold as compared with virus control or PKD1.KD ( Fig. 4a ). However, ducts generated by active PKD1 were neither as large nor as well developed as ducts obtained when metaplasia was induced with TGFα (compare Fig. 4b with Fig. 2b ). An average ductal area of 0.001 mm 2 was obtained after expression of active PKD1, which is approximately half the size of ducts obtained after TGFα treatment. This result indicates that although active PKD1 can drive the formation of ductal structures, additional TGFα-induced and probably PKD1-independent signalling is required for ducts to increase in size. 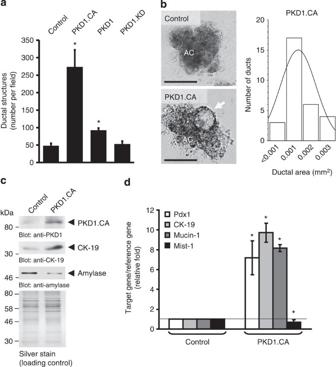There is also the possibility that the mutant does not fully reproduce the activity or localization of activated wild-type PKD1. Figure 4: Active PKD1 is sufficient to drive the formation of duct-like structures. (a) Primary acinar cells were isolated from mouse pancreas, infected with lentivirus harbouring control, wild-type PKD1, active PKD1 (PKD1.CA) or PKD1.KD, and seeded in collagen 3D culture. At day 7, ductal structures formed were quantified. (b–d) Primary acinar cells were isolated from mouse pancreas, infected with lentivirus harbouring control or active PKD1 (PKD1.CA) and seeded in collagen 3D culture. At day 7, ductal structures formed were photographed and ductal area (n=30) determined (b, scale bar, 100 μm). AC, acinar cells; the arrow indicates duct-like structure. In addition, ducts were isolated and analysed for markers of transdifferentiation (anti-CK-19 and anti-amylase) and expression of active PKD1, using western blotting (c), or for markers of acinar cell de- and transdifferentiation (Pdx1, Mist-1, CK-19 and mucin-1), using quantitative PCR (d). * Statistical significance (P<0.05; Student’st-test) as compared with control. Error bars (s.d.) were obtained from three experimental replicates. All experiments shown were performed at least three times with similar results. Figure 4: Active PKD1 is sufficient to drive the formation of duct-like structures. ( a ) Primary acinar cells were isolated from mouse pancreas, infected with lentivirus harbouring control, wild-type PKD1, active PKD1 (PKD1.CA) or PKD1.KD, and seeded in collagen 3D culture. At day 7, ductal structures formed were quantified. ( b – d ) Primary acinar cells were isolated from mouse pancreas, infected with lentivirus harbouring control or active PKD1 (PKD1.CA) and seeded in collagen 3D culture. At day 7, ductal structures formed were photographed and ductal area ( n =30) determined ( b , scale bar, 100 μm). AC, acinar cells; the arrow indicates duct-like structure. In addition, ducts were isolated and analysed for markers of transdifferentiation (anti-CK-19 and anti-amylase) and expression of active PKD1, using western blotting ( c ), or for markers of acinar cell de- and transdifferentiation (Pdx1, Mist-1, CK-19 and mucin-1), using quantitative PCR ( d ). * Statistical significance ( P <0.05; Student’s t -test) as compared with control. Error bars (s.d.) were obtained from three experimental replicates. All experiments shown were performed at least three times with similar results. Full size image Cells isolated from explant culture showed an increase in ductal markers (CK-19 and mucin-1) and a decrease in the acinar marker amylase at the protein and mRNA levels, when PKD1. CA was expressed ( Fig. 4c,d ). We also analysed samples for expression of Pdx1, an established marker for progenitor cells for endocrine and exocrine pancreatic cells. Pdx1 when expressed in the adult pancreas has been shown to drive de-differentiation of acinar cells to a more immature ductal cell type and to cause ADM [12] , [13] . Expression of active PKD1 upregulated Pdx1 approximately eightfold ( Fig. 4d ). The TGFα-Kras-PKD1 pathway acts through Notch The Notch signalling pathway has been established as a driver of acinar cell reprogramming to a ductal phenotype [21] , [27] , [30] . Therefore, using a Notch Signalling PCR array we analysed whether expression of active PKD1 in acinar cells affects the expression of Notch target genes, or genes that regulate Notch ( Fig. 5a ). Genes downregulated in their expression more than fourfold by active PKD1 included Cbl and Sel1l , both suppressors of Notch signalling. Genes upregulated more than fourfold in their expression by active PKD1 encode Adam10, Adam17 and MMP7, all proteinases that have been shown previously to mediate Notch activation [21] , [31] . In addition, we found upregulation of mRNA for the indirect Notch targets PPARγ ( Pparg ) and NF-κB1 ( Nfkb1 ) [32] , [33] . In this assay, active PKD1 also strongly upregulated mRNA expression of Hes-1, which is a direct target for Notch. Therefore, we next tested the involvement of the Notch pathway downstream of TGFα, Kras and PKD1. First, we tested whether Notch acts downstream of PKD1. We found that formation of ductal structures induced by active PKD1 can be effectively blocked when Notch1 was knocked down ( Fig. 5b ). This correlated with a decrease of expression of the Notch1 target Hes-1 ( Supplementary Fig. 4a ). Notch activity is regulated by cleavage at multiple levels [34] . Our data in Fig. 5a has shown that PKD1 upregulates proteinases that lead to S2 cleavage (Adam10 and Adam17). To mediate Notch activity, this first cleavage is followed by a second cleavage mediated by the γ-secretase complex (S3 cleavage). S3 cleavage leads to generation of the NICD (Notch intracellular domain) fragment that translocates to the nucleus [34] . Expression of active PKD1 in pancreatic acinar cells undergoing transdifferentiation indeed led to generation of NICD ( Fig. 5c ). Inhibiting S3 cleavage using the γ-secretase inhibitors DAPT and RO4929097 blocked PKD1-mediated formation of ductal structures, further indicating that PKD1 acts through activation of Notch ( Fig. 5d and Supplementary Fig. 4b ). Moreover, expression of the Notch targets Hes-1 and Hey-1 was decreased to basal levels in the presence of both γ-secretase inhibitors ( Fig. 5e ). As Notch is not the only target for γ-secretase, we also tested whether a S3-cleaved Notch fragment can drive ADM. To test this, we infected acinar cells with control virus or lentivirus harbouring NICD. We found that NICD induced the formation of ductal structures approximately twofold ( Fig. 5f ) and this correlated with the upregulation of the ductal marker CK-19, the dedifferentiation marker Pdx1 and the Notch target Hes-1 ( Supplementary Fig. 4c ). Next, we tested whether inhibition of γ-secretase also blocks ADM induced by the upstream regulators of PKD1, mutant Kras and TGFα. Acinar cells from LSL-Kras G12D mice were infected with control virus or virus harbouring cre recombinase to induce expression of Kras G12D . Expression of Kras G12D induced the expression of Notch target genes Hes-1 and Hey-1 ( Fig. 5g ), indicating that NICD is formed. Therefore, we next tested whether Kras G12D -driven ADM is blocked by DAPT or RO4929097. Both γ-secretase inhibitors decreased the formation of ductal structures by ~50% ( Fig. 5h ). Similar results were obtained when acinar cells were stimulated with TGFα. TGFα led to the upregulation of the Notch target genes Hes-1 and Hey-1 in a time-dependent manner, indicating that Notch is activated by S3 cleavage ( Fig. 5i ). Consequently, blocking of S3 cleavage by γ-secretase inhibitors blocked TGFα-mediated formation of ductal structures in 3D explant culture ( Fig. 5j ). In summary, our results show that PKD1 is necessary to mediate TGFα- and active Kras-induced reprogramming of pancreatic acinar cells to a duct-like phenotype that can give rise to PanIN lesions. Moreover, active PKD1, when expressed in acinar cells, is sufficient to initiate and drive this process. As one of the mechanism that is used by TGFα-Kras-PKD1 to drive this, we identify activation of the Notch signalling pathway ( Fig. 5k ). Increased TGFα and EGF signalling is frequently found in PDAC [2] , [3] . Similarly, activating Kras mutations are present in over 95% of all PDACs, and at a smaller percentage in PanIN lesions at all stages [1] . Transgenic expression of TGFα or active Kras in mouse pancreas resulted in ADM, convincingly demonstrating a role for these factors as inducers of the formation of duct-like cells and PanIN lesions in vivo [7] , [17] , [27] . Using an ex vivo explant 3D cell culture model in which primary pancreatic acinar cells are isolated and induced to undergo ADM and formation of ductal structures in the presence of growth factors such as EGF or TGFα [19] , [20] , [21] , [22] , [23] , we found that Kras is downstream of TGFα to drive ADM ( Fig. 2d,e ). This observation is important, as activating Kras mutations have been described as inducers of ADM in vivo [7] , but so far a role for active Kras in driving this process ex vivo was not well established. The fact that growth factors such as TGFα also use Kras to mediate ADM convincingly demonstrates that both pathways can converge at the level of Kras. PKD1 previously was implicated in pancreatic cancer, as it is overexpressed in patient samples [35] , whereas in normal pancreas PKD1 is not expressed in the exocrine cells [26] but has a role in insulin secretion of islets [36] . In PDAC cell lines, PKD1 contributes to cell proliferation and cell survival [35] , [37] , [38] , [39] , [40] , [41] , [42] , [43] . Moreover, it was recently shown that inhibition of PKD decreases orthotopic growth of pancreatic tumour cell lines in mice [37] . We show here that PKD1 signalling can contribute to very early events that alter pancreas cellular plasticity. Our data suggest that elevated levels of active PKD1 in pancreatic acinar cells are sufficient to drive the formation of duct-like cells ( Fig. 4 ). PKD1 is downstream of TGFα and active Kras to mediate formation of this cell type ( Fig. 2a–c and Fig. 3d,e ). Blockage of such signalling in vivo by knockout of PKD1 leads to decreased formation of PanIN lesions, which are based on this duct-like cell type ( Fig. 3f,g ). As specific small-molecule PKD inhibitors exist [37] , [41] , [44] , PKD1 is a promising new target to prevent ADM and further progression to PanIN lesions. Previously, it was shown that the transcription factor Prrx1b is induced during ADM, to upregulate expression of Sox9 (ref. 45 ). Sox9 in the presence of oncogenic Kras functions as an accelerator of formation of premalignant lesions [46] . Moreover, Sox9-deficient acinar cells expressing Kras G12D can undergo persistent ADM, but do not progress to PanINs [46] . As knockout of PKD1 in acinar cells also allows Kras G12D -mediated acinar cell metaplasia, but decreases further progression to PanIN lesions ( Fig. 3g ), a functional link between PKD1 and Sox9 may exist. Another possibility is a cross-talk of PKD1 signalling pathways with the phosphatidylinositol 3-kinase pathway. For example, it was shown that the knockout of Pten , a negative regulator of phosphatidylinositol 3-kinase signalling, leads to expression of Pdx1 and the Notch target gene Hes-1 (ref. 47 ), both markers for an undifferentiated epithelial phenotype [9] , [48] . Activation of PKD1 in pancreatic acinar cells also led to upregulation of Pdx1 and Hes-1. This suggested that PKD1 can promote dedifferentiation and reprogramming of pancreatic epithelial cells, which is believed to be one of the earliest events that can initiate pancreatic cancer. The Notch signalling pathway plays an important role during embryonic pancreas development, where it maintains an undifferentiated precursor cell type [48] . In the adult pancreas, the formation of duct-like cells induced by transgenic expression of TGFα is abolished when Notch activation is pharmacologically blocked [27] . Using explant cultures, it was further shown that Notch signalling can induce ADM and results in the accumulation of undifferentiated precursor cells [7] , [27] . Our results now suggest that PKD1 acts downstream of TGFα and Kras, to regulate the formation of duct-like cells via the Notch pathway. Specifically, we find that active PKD1 induced the expression of Adam10, Adam17 and MMP-7, all metalloproteinases that activate Notch directly by S2 cleavage and were previously linked to PDAC. For example, increased Adam17 mRNA expression and proteolytic activity was detected in pancreatic cancer cell lines, patient samples for chronic pancreatitis, as well as tissues with PanIN3 lesions or PDAC [31] , [49] . A similar result was found for Adam10 in human tissue samples of chronic pancreatitis and PDAC [50] . Direct cleavage of Notch by MMP-7 leads to its activation and contributes to acinar-to-ductal transdifferentiation [21] . Our data further indicate that active PKD1 also leads to formation of an active cytoplasmic domain (NICD), a final activation step that is mediated through S3 cleavage by γ-secretases ( Fig. 5c ). Consequently, treatment with the γ-secretase inhibitors DAPT or RO4929097, which block Notch S3 cleavage, led to a decrease of PKD1-, TGFα- and Kras-mediated expression of the Notch target genes Hes-1 and Hey-1 , as well as decreased formation of ductal structures ( Fig. 5d–j ). Increased Hes-1 expression is a bona fide marker for development of pancreatic cancer, as it was found to be upregulated in preneoplastic lesions and pancreatic cancers in humans and mice [2] , [7] . In summary, understanding the signalling pathways that regulate the reprogramming of acinar cells to a duct-like cell type that can give rise to PanIN lesions is important for risk prognosis or early diagnosis of pancreatic cancer. Such knowledge may be used for identifying targetable signalling molecules that allow prevention of progression, and possibly phenotype reversion as well. Here we identify PKD1 as a key signalling protein downstream of EGF-R and Kras, which drives the formation of such duct-like cells and is pharmacologically targetable by novel small-molecule PKD-specific inhibitors. Antibodies and reagents The anti-amylase and anti-β-actin antibodies were from Sigma-Aldrich (St Louis, MO), anti-CK-19 antibody from Leica Microsystems (Buffalo Grove, IL), anti-claudin-18 antibody from Invitrogen (Carlsbad, CA), anti-Ras antibody from Epitomics (Burlingame, CA), anti-GST and anti-green fluorescent protein (GFP) from Santa Cruz (Santa Cruz, CA), anti-activated Notch1 antibody from Abcam (Cambridge, MA), anti-PKD1 from Antibodies-online Inc. (Atlanta, GA), anti-PKD2 from Acris Antibodies (San Diego, CA), anti-PKD3 antibody from Bethyl Laboratories (Montgometry, TX) and anti-pS744/748-PKD antibodies from Cell Signaling Technology (Danvers, MA) or Abcam. Recombinant human TGFα was purchased from Chemicon (Billerica, MA) and R&D Systems (Minneapolis, MN). Dexamethasone was from Sigma-Aldrich, soybean trypsin inhibitor and collagenase I from Affymetrix (Santa Clara, CA). Phenol red-free Matrigel and rat tail collagen I were from BD Biosciences (San Diego, CA). Hoechst 33342 was purchased from Invitrogen (Grand Island, NY). The PKD inhibitor CRT0066101 was from TOCRIS (Ellisville, MO) and kb-NB-142-70 was described previously [51] . The γ-secretase inhibitors DAPT and RO4929097 were from Cellagen Technology (San Diego, CA). Viral constructs Adenovirus to express Cre recombinase (Adeno-Cre and Ad-CMV-Cre) was purchased from Vector Biolabs (Philadelphia, PA). A lentiviral construct (plasmid 17623, EF.hICN1.CMV.GFP) to express the intracellular domain of Notch (NICD) was from Addgene (Cambridge, MA). pLenti6.3/V5-GFP-PKD1, pLenti6.3/V5-GFP-PKD1.CA or pLenti6.3/V5-GFP-PKD1.KD were generated by amplifying previously described GFP-tagged human PKD1, PKD1.S738E.S742E or PKD1.K612W, using the following primers: 5′-CTGGATCCATGAGCGCCCCTCCGGTC-3′ and 5′-CCGCTCGAGTTACTTGTACAGCTCGTC-3′. The amplicon was inserted into pLenti6.3/V5-TOPO vector (Invitrogen) via TOPO cloning. pLenti6.3/V5-Flag-TdTomato-Kras G12V was generated by amplifying a Flag-Kras G12V mutant using 5′-GCGGGATCCATGGACTATAAGGACGATGATGACAAAACTGAATATAAACTTGTGGTAGTT-3′ and 5′-GCGACTAGTCATAAATTACACACTTTGTCTTTGA-3′ as primers. The amplicon was inserted into pLenti6.3/V5-TOPO vector (Invitrogen) via TOPO cloning. TdTomato was amplified from pRSET-B-tdTomato (gift from R. Tsien, UCSD), using 5′-AAGGATCCGCAATGGTGAGCAAGGGC-3′ and 5′-TAGGATCCCTTGTACAGCTCGTC-3′ as primers and then inserted into pLenti6.3/V5-Flag-Kras G12V via BamHI restriction sites. The obtained plasmid was confirmed by PCR for the correct orientation of TdTomato. Lentiviral plasmids to knock down murine PKD1, Kras or Notch1 were purchased from Sigma-Aldrich. The hairpin sequences for mPKD1-shRNA#1 and mPKD1-shRNA#2 were 5′-CCGGGAGTGTTTGTTGTTATGGAAACTCGAGTTTCCATAACAACAAACACTCTTTTT-3′ and 5′-CCGGCCTTCAGCTTTAACTCCCGTTCTCGAGAACGGGAGTTAAAGCTGAAGGTTTTT-3′, respectively. The hairpin sequences for murine Kras-shRNA were 5′-CCGGCAAGTAGTAATTGATGGAGAACTCGAGTTCTCCATCAATTACTACTTGTTTTTG-3′ (labeled as Kras-shRNA#1) and 5′-CCGGGTGTTGACGATGCCTTCTATACTCGAGTATAGAAGGCATCGTCAACACTTTTTG-3′ (labelled as Kras-shRNA#2). The hairpin sequences for murine Notch1-shRNA were 5′-CCGGGCCAGGTTATGAAGGTGTATACTCGAGTATACACCTTCATAACCTGGCTTTTT-3′ (labelled as mNotch1-shRNA#1) and 5′-CCGGGCAGATGATCTTCCCGTACTACTCGAGTAGTACGGGAAGATCATCTGCTTTTT-3′ (labelled as mNotch-shRNA#2). Genetic animal models MT-TGFα mice in a C57Bl/6 background were kept on 10 mM ZnSO 4 in the drinking water to induce the TGFα transgene. LSL-Kras G12D mice (obtained from the NCI Mouse Repository; MMHCC) were crossed with p48 cre mice (a gift from Dr Pinku Mukherjee, University of North Carolina) to generate bi-transgenic p48 cre ;LSL-Kras G12D mice. A detailed scheme of the strategy to generate mice with an acinar cell-specific knockout of PKD1 as well as a representative genotyping and analysis are shown in Supplementary Fig. 3b,c,f . The PKD1 targeted allele (PKD1 gene locus on homologous recombination of the targeting vector) was crossed into a mouse line ubiquitously expressing Flip, to obtain the mouse line with PKD1 floxed allele. PKD1 floxed mice were crossed with p48 cre mice to obtain mice with acinar cell-specific knockout of PKD1 (p48 cre ;PKD1 −/− mice). Next, LSL-Kras G12D mice were crossed with PKD1 fl/fl mice to generate LSL-Kras G12D ;PKD1 fl/fl mice. Eventually, p48 cre ;PKD1 −/− mice were crossed with LSL-Kras G12D ;PKD1 fl/fl mice to obtain p48 cre ;Kras G12D ;PKD1 −/− mice. All animal experiments performed were in compliance with ethical regulations and were approved by the Mayo Clinic Institutional Animal Care and Use Committee. Isolation of primary pancreatic acinar cells and 3D culture The procedure to isolate primary pancreatic acinar cells was described in detail previously [18] . In brief, the pancreas was removed, washed twice with ice-cold Hank’s balanced salt solution (HBSS) media, minced into 1–5 mm pieces and digested with collagenase I (37 °C, shaker). Collagen digestion was stopped by adding an equal volume of ice-cold HBSS media containing 5% fetal bovine serum (FBS). The digested pancreatic pieces were washed twice with HBSS media containing 5% FBS and then pipetted through 500 μm and then 105 μm meshes. The supernatant of the cell suspension containing acinar cells was added dropwise to 20 ml HBSS containing 30% FBS. Acinar cells were then pelleted (1,000 r.p.m., 2 min at 4 °C) and re-suspended in 10 ml Waymouth complete media (1% FBS, 0.1 mg ml −1 trypsin inhibitor, 1 μg ml −1 dexamethasone). For the 3D explant culture [21] , [22] , [23] , cell culture plates were coated with collagen I in Waymouth media without supplements. Isolated primary pancreatic acinar cells were added as a mixture with collagen I/Waymouth media on the top of this layer. Further, Waymouth complete media was added on top of the cell/gel mixture, replaced the following day and then every other day. When growth factors or inhibitors were added, the compound of interest was added to both the cell/gel mixture and the media on top. To express proteins using adeno- or lentivirus, acinar cells were infected with virus of interest and incubated for 3–5 h before embedding in the collagen/Waymouth media mixture. At day 5–7 (dependent on time course of duct formation), numbers of ducts were counted under a microscope and photos were taken to document structures. The area of ducts was measured using Image J software and StatsDirect (StatsDirect Ltd; http://www.statsdirect.com ) to obtain a distribution curve. Determination of cell viability Cellular viability was assessed using Hoechst 33342 without fixation step (staining of cells that are alive). Therefore, the media on top of the 3D culture were removed, the mixture of cell/collagen was rinsed twice with PBS and incubated with Hoechst 33342 (2.5 μg ml −1 in PBS) at 37 °C for 30 min. After three washes in PBS, Hoechst 33342-stained cells were visualized using a DAPI (4,6-diamidino-2-phenylindole) filter with an Olympus IX71 fluorescent microscope, × 10 magnification and DP70 digital camera. Measurement of Ras activity Ras activity was assessed using Raf-1-RBD pull-down assays. In brief, freshly isolated acinar cells were treated with 100 ng ml −1 TGFα for indicated times. Cells were lysed with Buffer A (50 mM Tris/HCl pH 7.4, 1% Triton X-100, 150 mM NaCl, 5 mM EDTA) plus protease inhibitor cocktail (Sigma-Aldrich). Clarified cellular lysates were incubated with 20 μg GST-Raf-1-RBD (aa1-149) for 90 min at 4 °C, followed by three washes with Buffer A. Samples were run on SDS–PAGE, transferred to nitrocellulose membrane and analysed for Ras (anti-Ras antibody). Input was controlled by staining with α-GST antibodies (GST-Raf-1-RBD input) or by staining of lysates for total Kras or β-actin. Immunohistochemistry Slides were de-paraffinized (1 h, 60 °C), de-waxed in xylene (five times, 4 min) and gradually re-hydrated with ethanol (100%, 95%, 75%, each two times, 3 min). Re-hydrated samples were rinsed in water and subjected to antigen retrieval in 10 mM sodium citrate buffer pH 6.0 (DAKO, Carpinteria, CA). Slides were treated with 3% H 2 O 2 (5 min) to reduce endogenous peroxidase activity, washed with PBS containing 0.5% Tween 20 and blocked with protein block serum-free solution (DAKO) for 5 min at room temperature (RT). Samples were stained with haematoxylin and eosin, Alcian Blue, anti-claudin-18 antibody (1:1,000), anti-PKD1 antibody (1:100), anti-PKD2 antibody (1:200), anti-PKD3 antibody (1:200), or anti-pS744/748-PKD antibody (Abcam) at a dilution of 1:50 in Antibody Diluent Background Reducing Solution (DAKO) and visualized using the Envision Plus Dual Labeled Polymer Kit (DAKO), according to the manufacturer’s instructions. Images were captured using the ScanScope XT scanner and ImageScope software (Aperio, Vista, CA). Immunostaining and confocal microscope imaging Freshly isolated acinar cells were plated in phenol red-free Matrigel on top of a pre-coated chamber glass slide. Phenol red-free Waymouth complete media was added to the top of the polymerized Matrigel/acinar cell mixture. After duct formation, cells were fixed with 4% formaldehyde in PBS for 20 min at RT, permeabilized with 0.5% Triton X-100 in PBS for 30 min at RT, washed three times with PBS and blocked with 10% goat serum in PBS cells for 1 h at RT. Samples were incubated with primary antibodies (anti-PKD1 at 1:500, anti-CK-19 at 1:200 and anti-amylase at 1:300) at 4 °C overnight. Samples were washed three times with PBS containing 0.2% Triton X-100. Secondary antibodies (Alexa Fluor 546 goat-anti-rabbit from Invitrogen at 1:500) were added for 1 h at RT. Samples were washed three times with PBS. Images were captured using a LSM 510META confocal laser scanning microscope (Zeiss) with a × 20 objective lens. RNA isolation and quantitative real-time PCR Cells were harvested from explant 3D collagen culture by digestion in 1 mg ml −1 collagenase solution at 37 °C for 30 min on a shaker. Cells were washed once with HBSS and twice with PBS, and total RNA isolation was performed using the miRCURY RNA isolation kit (Exiqon, Woburn, MA) and the TURBO DNA-free kit (Ambion, Austin, TX), to eliminate residual genomic DNA. mRNA of interest was assessed using a two-step quantitative reverse transcriptase-mediated real-time PCR method. Equal amount of total RNA was converted to complementary DNA by the high-capacity cDNA reverse-transcriptase kit (Applied Biosystems, Bedford, MA). Quantitative PCR was performed in a 7900HT Fast real-time thermocycler (Applied Biosystems) using the TaqMan Universal PCR master mix (Applied Biosystems) with probe/primer sets and the following thermocycler programme: 95 °C for 20 s, 40 cycles of 95 °C for 1 s and 60 °C for 20 s. All probe/primer sets were purchased from Applied Biosystems (PKD1: Mm00435790_m1; Pdx1: Mm00435565_m1; CK-19: Mm00492980_m1; mucin-1: Mm00449604_m1; Mist-1: Mm00627532_s1; Hes-1: Mm01342805_m1; Hey-1: Mm00468865_m1; glyceraldehyde 3-phosphate dehydrogenase: Mm99999915_g1; 18S rRNA: Hs99999901_s1). The amplification data were collected by a Prism 7900 sequence detector and analysed with Sequence Detection System software (Applied Biosystems). Data were normalized to murine glyceraldehyde 3-phosphate dehydrogenase or 18s RNA, and mRNA abundance was calculated using the ΔΔ C T method. Quantitative real-time PCR with the mouse Notch Signaling Targets PCR Array (SA Biosciences, Frederick, MD) was carried out according to the manufacturer’s instructions and data were analysed with the web-based RT 2 Profiler PCR Array software (SA Biosciences). Cellular extracts and immunoblotting Cells were harvested from explant 3D collagen culture by digestion in 1 mg ml −1 collagenase solution at 37 °C for 30 min on a shaker. Cells were washed once with HBSS, twice with PBS and lysed in Buffer A (50 mM Tris/HCl pH 7.4, 1% Triton X-100, 150 mM NaCl, 5 mM EDTA) supplemented with protease inhibitor cocktail (Sigma). Lysates were incubated on ice for 30 min, centrifuged (13,000 r.p.m., 15 min, 4 °C) and supernatants were subjected to SDS–PAGE. Gels were either stained by silver gel staining (Pierce silver stain kit, Thermo Scientific) or resolved proteins were transferred to nitrocellulose membranes. Membranes were blocked with 5% BSA in TBST (50 mM Tris/HCl, pH 7.4, 150 mM NaCl, 0.1% Tween 20) and incubated with primary antibodies of interest in 5% BSA in TBST overnight at 4 °C, and then with horseradish peroxidase-conjugated secondary antibodies for 1 h at RT. Samples were visualized with enhanced chemiluminescence and X-ray film ( Supplementary Fig. 5 ). Statistical analysis Data are presented as mean±s.d. P -values were acquired with the Student’s t -test, using Graph Pad software and P <0.05 is considered statistically significant. How to cite this article: Liou, G.-Y. et al. Protein kinase D1 drives pancreatic acinar cell reprogramming and progression to intraepithelial neoplasia. Nat. Commun. 6:6200 doi: 10.1038/ncomms7200 (2015).